Evidence for the stress-linked immunocompetence handicap hypothesis in humans Secondary sexual traits that develop under the action of testosterone, such as masculine human male facial characteristics, have been proposed to signal the strength of the immune system due to the sex hormone's immunosuppressive action. Recent work has suggested that glucocorticoid stress hormones may also influence expression of such sexual signals due to their effects on immune function. Precise roles, however, remain unclear. Here we show positive relationships between testosterone, facial attractiveness and immune function (antibody response to a hepatitis B vaccine) in human males, and present some preliminary evidence that these relationships are moderated by naturally co-occurring cortisol (a glucocorticoid stress hormone involved in the fight-or-flight response). We conclude that our results provide support for a role of glucocorticoids in hormonally mediated sexual selection. Testosterone-dependent traits have been proposed to provide an honest signal of male immune function due to the sex hormone's immunosuppressive effects [1] . A review of cross-species data, however, has demonstrated inconsistent effects of testosterone (T) on immune function [2] , and glucocorticoids have been proposed to contribue to this complexity [3] , [4] . These stress hormones modulate the immune system [5] and expression of secondary sexual traits [6] and they may interact with T in effects on both [7] , [8] , [9] . Precise roles in sexual selection, however, remain unclear due to the reliance of extant tests on artificial elevation of T, such that interactions with glucocorticoids may result from the stressful implantation procedure or from T levels elevated beyond an individual's natural range [7] . Sexually dimorphic characteristics in the human male face are T-dependent [10] , [11] , and female preferences for these have been interpreted as a strategy to secure heritable immunocompetence for offspring [12] , [13] . Here we demonstrate positive relationships between T, facial attractiveness and immune response to a hepatitis B vaccine, and present some evidence that these relationships are moderated by naturally co-occurring cortisol (C). Our results are the first to show that human female face preferences are correlated directly with a measure of male immune function, and to provide some preliminary evidence of a possible moderating role of glucocorticoids in relationships between T, secondary sexual trait expression and immune function. We anticipate that our findings will provide a platform for the development of a more powerful model of hormonally mediated sexual selection that incorporates specific functions of glucocorticoids. Sample characteristics A total of 74 males (age: 23.12 (3.89)) were recruited from the University, and Transportation College, of Daugavpils, Latvia. Use of human subjects complied with the regulations of the University of Daugavpils and the Declaration of Helsinki. We assessed T, C and anti-hepatitis B surface antigen (anti-HBsAg) levels from 10 ml of venous blood collected between 0900 and 1100 h, approximately 30 min before and 1 month after the first dose of a hepatitis B vaccine. Anti-HBsAg, T and C were measured using commercially available immunoassays. No participant expressed anti-HBsAg before vaccination (post-vaccination: 9.53 (13.68) mIU ml −1 ), 16 participants (21.6%) did not produce antibodies (non-seroconverters; levels consistent with previous research [14] ) and 27 participants (36.5%) were seroprotected (produced ≥10 mIU ml −1 of anti-HBsAg). T levels were attained for all participants (10.68 (2.85) nmol l −1 ), and C levels were attained for a sub-sample of 62 participants (463.43 (152.28) nmol l −1 ). T and C showed strong consistency across samples (intraclass correlation coefficients (3, 1) were 0.81 and 0.91, respectively), so we calculated means for each participant. Facial photographs were collected under standardized lighting conditions with neutral expression, normalized on interpupillary distance and rated by 94 female students of the University of Daugavpils (age: 20 (1.89)) from −5 (very unattractive) to +5 (very attractive). Inter-rater reliability was high (Cronbach's alpha=0.97), so we computed the mean attractiveness scores for each male participant. Relationships between T, C, anti-HBsAg and attractiveness A Box–Cox transformation was applied to anti-HBsAg to obtain a normal distribution (Kolmogorov–Smirnov: P =0.057; skewness= −0.39). There was no significant difference between seroconverters (SC) and non-SCs (NSC) in C (SC: 459.3 (157.25) nmol l −1 ; NSC: 477.58 (138.33) nmol l −1 ; F (1, 61) =0.15, P =0.696, two-tailed), but there were significant differences in T (SC: 11.43 (2.63) nmol l −1 ; NSC: 7.94 (1.75) nmol l −1 ; F (1, 73) =25.1, P <0.001) and attractiveness (SC: −1.56 (1.19); NSC: −2.58 (0.57); F (1, 73) =10.83, P =0.002, two-tailed). We therefore conducted all analyses in the full sample and the SC sub-sample. 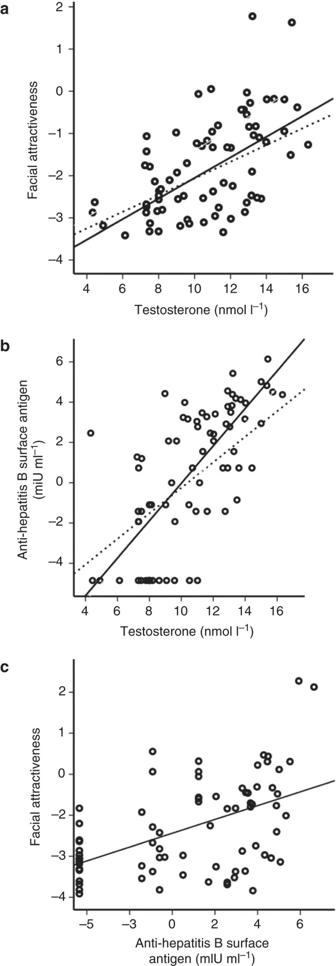Figure 1: Relationships between testosterone and antibody levels compared with attractiveness. Relationships between testosterone (nmol l−1) and (a) facial attractiveness (n=74,P<0.001) and (b) anti-hepatitis B surface antigen (mIU ml−1; Box–Cox transformed;n=74,P<0.001) showing moderating effects of cortisol (for a subsample of 62 participants for whom cortisol measurements were available; bold lines: cortisol below the median; broken lines: cortisol above the median) and between (c) anti-hepatitis B surface antigen (mIU ml−1) and facial attractiveness (n=74,P<0.001). We used linear regression models to test for bivariate relationships between T, C, a T×C interaction term, anti-HBsAg and attractiveness (all two-tailed, Table 1 ). T predicted attractiveness (full sample: Adj R 2 =0.31, F (1, 73) =34.08, P <0.001, Fig. 1a ; SC: Adj R 2 =0.21, F (1, 57) =16.2, P <0.001) and anti-HBsAg levels (full sample: Adj R 2 =0.45, F (1, 73) =61.21, P <.001, Fig. 1b ; SC: Adj R 2 =0.3, F (1, 57) =25.38, P <0.001), such that males with high T had higher facial attractiveness ratings and anti-HBsAg levels than those with low T. Anti-HBsAg levels predicted attractiveness (full sample: Adj R 2 =0.24, F (1, 73) =23.67, P <0.001, Fig. 1c ; SC: Adj R 2 =0.13, F (1, 57) =9.84, P =0.003), such that the faces of males with a strong immune response to vaccination were perceived as more attractive by females than those with a weaker response. The T×C interaction term predicted attractiveness and anti-HBsAg only in the full sample (attractiveness: Adj R 2 =0.05, F (1, 61) =4.27, P =0.043, Fig. 1a ; SC: Adj R 2 =0.01, F (1, 47) =1.31, P =0.259; anti-HBsAg: Adj R 2 =0.11, F (1, 61) =8.32, P =0.005, Fig. 1b ; SC: Adj R 2 =0.04, F (1, 47) =3.01, P =0.089). As T and T×C were significant predictors of both attractiveness and anti-HBsAg in the full sample, and anti-HBsAg was a significant predictor of attractiveness, multiple linear regression models were constructed to determine whether anti-HBsAg levels mediated relationships between T and attractiveness, and T×C and attractiveness. Table 1 shows that anti-HBsAg mediated the relationship between T×C and attractiveness (full sample: Adj R 2 =0.27, F (2, 61) =12.21, P <0.001; T×C: β =0.08, P =0.494; anti-HBsAg: β =0.51, P <0.001), but not the relationship between T and attractiveness. Table 1 β values for the bivariate relationships. Full size table Figure 1: Relationships between testosterone and antibody levels compared with attractiveness. Relationships between testosterone (nmol l −1 ) and ( a ) facial attractiveness ( n =74, P <0.001) and ( b ) anti-hepatitis B surface antigen (mIU ml −1 ; Box–Cox transformed; n =74, P <0.001) showing moderating effects of cortisol (for a subsample of 62 participants for whom cortisol measurements were available; bold lines: cortisol below the median; broken lines: cortisol above the median) and between ( c ) anti-hepatitis B surface antigen (mIU ml −1 ) and facial attractiveness ( n =74, P <0.001). Full size image Significant relationships in the full sample remained in the SC sample, with the exception of T×C with attractiveness and anti-HBsAg. Furthermore, when anti-HBsAg was dichotomized using a median split and entered as the dependent variable in binary logistic regression models, T (Nagelkerke R 2 =0.33, Wald=15.12, P <0.001, two-tailed) remained as a significant predictor and T×C showed a trend towards significance (Nagelkerke R 2 =0.08, Wald=3.4, P =0.065, two-tailed), and there was a significant difference in attractiveness between the two groups (low anti-HBsAg: −2.11 (0.96); high anti-HBsAg: −1.45 (1.27); F (1, 72) =6.51, P =0.013, two-tailed). Two participants received facial attractiveness ratings that were above the mean+2 s.d. ( Fig. 1a and c ). All significant relationships remained when these participants were excluded from the analyses, with the exception of that between the T×C interaction term and attractiveness (Adj R 2 =0.02, F (1, 60) =2.22, P =0.141, two-tailed). Our results provide the first evidence that women's preferences for male faces are correlated with male immunocompetence and for a consistent interaction between T and C on immune function and facial attractiveness. This provides support for a stress-linked version of the immunocompetence handicap model of sexual selection and demonstrates that the role of glucocorticoids was such that positive relationships between T and immune response to a vaccine, and T and facial attractiveness, were stronger in those males with low C. Furthermore, the interaction between T and C in effects on attractiveness was mediated by immune function, whereas the relationship between T and attractiveness was not. This suggests that those T-related traits that interact with C are linked to immunocompetence, but that T may also be related to additional traits that contribute to attractiveness such as ability to acquire resources [15] . Although we exert caution in interpreting the positive relationship between naturally occurring T and immune function as support for an immunocompetence handicap model (it is possible to predict positive or negative relationships depending upon the quality and condition of males in the sample [16] ), our results provide some evidence of a moderating role of glucocorticoids in data collected using non-invasive techniques that are unlikely to have resulted in artificial elevation of T or C. Glucocorticoids have been proposed to mediate pathways between T, immune function and secondary sexual ornamentation [4] (for example, through competition for binding sites [17] ). Lack of consistency in the nature of the relationship between T and glucocorticoids [7] , and our failure to demonstrate such mediation here suggest that this is not the case. Our results, instead, suggest a moderating role of C, such that the relationships of the immunocompetence handicap model of sexual selection may be contingent upon co-occurring levels of glucocorticoids. This may explain inconsistencies in relationships between T and measures of immune function across the samples [2] . To interpret the interaction between T and C, it is necessary to determine whether our measure of morning C is a proxy of experience of current stressors [18] or individual differences in traits such as baseline C or dimensions of the physiological response to stress. In the former, the effects of T on facial appearance and immune function are transient and dependent upon the current level of stress experienced by the individual, whereas in the latter, there may be an optimal baseline level of C or response to stress that bears minimum costs to immune function or sexual signalling [7] , [8] , [9] . Tests of the effects of T on immunity and appearance under periods of high and low stress, and identification of the effects of dimensions of the C response to a stressor and baseline levels collected from multiple points in C's natural diurnal cycle on the relationships of interest, will enable development of a model of specific functions of glucocorticoids in sexual selection. We found T and C to interact in their effects on antibody response to a vaccination, such that the positive relationship between T and immune response was stronger in males with low C. We found a consistent, but weak, interaction between T and C on facial attractiveness. Facial cues to combinations to T and C may be subtle, and more robust relationships may be detected in a larger sample with greater variance or by constructing facial composites that are designed to differ in cues to the hormones [9] . Both relationships lost significance when participants who did not produce antibodies were excluded from analyses. Although interactions between sex and stress hormones have been reported in previous studies, the nature of these results has been inconsistent. Male zebra finch ( Taeniopygia guttata ) with the highest titres of T and corticosterone, for example, showed the strongest secondary response to diptheria [7] , whereas no such interaction was found in the Japanese quail ( Coturnix japonica ) [19] . Such discrepancies may arise from differences in exposure to stress or socioecological conditions across species and samples. Such inconsistency is also evident in tests across human societies. In studies conducted in the UK, women typically express preferences for the faces of males with cues to low T [12] , [13] , and an interaction has been shown between T and C on facial attractiveness, such that T increases attractiveness in males with high C, but decreases attractiveness in those with low C [9] . The current results from a Latvian sample show a positive relationship between T and facial attractiveness that was strongest in males with low C. Recent research has shown societal level measures of health to influence women's preferences for cues to T in the male face [13] , meaning that societal level factors may underpin differences in the preferences of women from the UK and Latvia. Tests of relationships across species, societies and contexts will further inform as to the traits signalled by combinations of sex and stress hormones. Although antibody response to vaccination provides an accurate measure of response across the immune system [20] , future tests should assess different arms of the immune response to evaluate trade-offs between, for example, cellular and humoral immunity. In addition, tests should be conducted in samples of males at different life stages (for example, adolescence and older adulthood) to determine whether the relationships reported here are specific to the high T levels typical of early adulthood [21] . To conclude, our results provide support for the stress-linked immunocompetence handicap model of sexual selection. Positive relationships between T, immune response to a vaccine, and facial attractiveness were stronger in males with low naturally co-occurring C, implicating a moderating role of glucocorticoids in hormonally mediated sexual selection. The nature of traits that are signaled by combinations of sex and stress hormones can be tested by systematic investigation of these relationships across species and contexts. Hepatitis B vaccine The hepatitis B vaccine is delivered intramuscularly using a three-dose protocol over 6 months and contains hepatitis B surface antigen derived from yeast cells. All participants received the Engerix B vaccine manufactured by Glaxosmithkline [22] . Antibody response provides an estimate of total immune function due to reliance on interactions between multiple arms of the immune system [20] , and response to the hepatitis B vaccine was appropriate because of low prior exposure in the target population [23] and correlations between antibody response to the vaccine, disease resistance [24] and psychological measures [25] . Levels of anti-HBsAg were assessed at the E. Gulbis Laboratory, Daugavpils, Latvia, using an in-house microparticle enzyme immunoassay (AxSYM®, Abbott Laboratories) and commercially available kits (AUSAB®, Abbott Laboratories [26] ). Blood samples were centrifuged and the separated serum frozen at −80 °C until analysis. Serum was incubated with microparticles coated with recombinant human HBsAg at room temperature for 24 h. The beads were then incubated with HBsAg conjugated to biotin and rabbit anti-biotin antibody conjugated with horseradish peroxidase, allowing absorbency of control and test samples to be measured. Mean intra-assay CV was 2.9%, the lower level of detection was 2 mIU ml −1 and the analytical range was 2–1000 mIU ml −1 . The range of anti-HBsAg in the sample was 0–73 mIU ml −1 . Testosterone Testosterone was assessed in the same laboratory using an in-house competitive chemoluminescent enzyme immunoassay with commercially available kits (Immulite ® 2000 Total Testosterone [27] ). Serum samples were incubated for 60 min at 370 °C with an alkaline phosphatase-labeled reagent and polystyrene beads coated with polyclonal rabbit antibody. Unbound material was removed by centrifugal wash, and bound quantities were measured using a specific chemoluminescent substrate (a phosphate ester of adamantyl dioxetane). Immulite ® 2000 Total Testosterone quality control samples were included to assess the assay reliability. Mean intra-assay CV was 9.6%, the method lower limit of detection was 0.694 nmol l −1 (manufacturer's standard: 0.3 nmol l −1 (ref. 27 )) and the analytical range was 0.694–55.52 nmol l −1 . The range of T in the sample (4–16.3 nmol l −1 ) was lower than published reference ranges for young adult males (for example, 10.4–41.6 nmol l −1 (ref. 28 )). This is likely to be due to a negative bias and/or underestimation of T reported for the Immulite ® platform [29] and is unlikely to have influenced our assessment of inter-individual variation in T. Cortisol C levels were determined in the same laboratory using Immulite ® 2000 Cortisol, following the procedure described above [27] , for a subset of the sample ( n =62). Cortisol was not assessed for the remaining 12 participants due to insufficient quantities of remaining serum. In this case, the alkaline phosphatase-labelled reagent was conjugated to C, and polystyrene beads were coated with polyclonal rabbit anti-C. Immulite ® 2000 Cortisol quality control samples were included to assess assay reliability. Mean intra-assay CV was 6.6%, the method lower limit of detection was 27 nmol l −1 (manufacturer's standard: 5.5 nmol l −1 (ref. 27 )) and the analytical range was 28–1380 nmol l −1 . The range of C in the sample (205–759 nmol l −1 ) extended above published reference ranges (140–690 nmol l −1 ) [28] , which is likely to be due to our collection of samples in the morning, which coincides with a natural peak in the diurnal fluctuation of C [30] . How to cite this article: Rantala, M. J. et al . Evidence for the stress-linked immunocompetence handicap hypothesis in humans. Nat. Commun. 3:694 doi: 10.1038/ncomms1696 (2012).